Pirt reduces bladder overactivity by inhibiting purinergic receptor P2X3 Pirt is a transmembrane protein predominantly expressed in peripheral neurons. However, the physiological and pathological roles of Pirt in hollow viscus are largely unknown. Here we show that Pirt deficiency in mice causes bladder overactivity. The density of α,β-meATP-induced currents is significantly reinforced in Pirt-deficient dorsal root ganglion (DRG) neurons. Pirt and P2X3 receptor co-localize in bladder nerve fibres and heterologous Pirt expression significantly reduces P2X3-mediated currents. Pirt interacts with P2X3 through the N-terminal 14 amino-acid residues. TAT-conjugated Pirt N14 peptide (Pirt N14 ) is sufficient to inhibit P2X3 activation in bladder DRG neurons and to alleviate bladder overactivity in Pirt −/− mice. Pirt expression is decreased in the bladder of cyclophosphamide (CYP)-treated mice, a commonly used model of bladder overactivity. Importantly, Pirt N14 administration reduces the frequency of bladder voiding and restores the voided volume of CYP-treated mice. Therefore, our results demonstrate that Pirt is an endogenous regulator of P2X3 in bladder function. Urgency and frequency are common symptoms of bladder overactivity, including neurogenic bladder, overactive bladder, bladder outlet obstruction and interstitial cystitis. According to a survey of 12,572 women, up to 6.5% met the symptom criteria for bladder pain syndrome/interstitial cystitis in the United States [1] . Overactive bladder syndrome affects 66 million people in the European Union, and the incidence of overactive bladder syndrome is up to 40% of individuals over the age of 70 in Europe [2] . In Asia, it is reported that over 22.9% of the population over 30 years of age in Korea are suffering from overactive bladder, and their health-related quality of life has been severely affected [3] . Activity in the bladder is initiated by muscarinic receptor stimulation in smooth muscle, and currently, antimuscarinic drugs are the first-line of treatment [4] . However, those drugs only have a slightly better effect than placebo, and the side effects and the lack of sufficient efficacy cause poor patient compliance [5] . Therefore, it is important and necessary to explore the mechanisms of bladder overactivity to develop new therapeutic strategies. The bladder wall has three layers—the urothelium, the suburothelial layer and the muscle layer. In response to physical and chemical stimulation, the urothelium releases several substances, including acetylcholine, ATP, prostaglandins and so on [6] , [7] , [8] . These chemical agents modify afferent nerve activity and sensation in the suburothelial layer and in the muscle layer [2] . P2X2/3 channels are ATP receptors and are expressed on bladder afferent fibres. During bladder inflammation, the amount of ATP from the urothelium is increased [9] . ATP released from the urothelium can interact with P2X2/3 receptors and enhance the excitability of afferent bladder nerves [10] . However, P2X3-null mice exhibit a marked urinary bladder hyporeflexia characterized by decreased voiding frequency and increased bladder capacity [11] . These reports suggest that the P2X3 receptors of afferent nerves play a crucial role in bladder control. However, the regulation of P2X3 receptors on bladder afferent nerves during physiological or pathological states is still unclear. Pirt is a small transmembrane protein and is expressed predominantly in peripheral nociceptive neurons, particularly in dorsal root ganglia neurons. Pirt -knockout mice displayed reduced sensitivity to noxious heat [12] . Further work revealed that Pirt is an endogenous regulator for TRPV1 and TRPM8 (refs 12 , 13 ). In the present study, we demonstrate that Pirt regulates bladder voiding via the inhibition of purinergic receptor P2X3 and that a peptide derived from Pirt has inhibiting effects on bladder overactivity. Pirt deficit causes bladder overactivity Pirt is expressed specifically in the peripheral nervous system [12] and may play a role in the regulation of internal organ functions. To examine the role of Pirt in bladder voiding, we measured the micturition frequencies and the void volumes of Pirt null ( Pirt −/− ) mice. As shown in Fig. 1 , the voiding contraction of Pirt −/− mice was 36.0±3.1 times during 15 min of intravesical saline perfusion, while that of wild-type (WT) mice was 25.1±2.0 times ( P =0.00856, two-tailed unpaired Student’s t -test). Furthermore, the mean void volume of Pirt −/− mice was 0.036±0.004 ml, while that of WT mice was 0.059±0.005 ml ( P =0.00672, two-tailed unpaired Student’s t -test). The increased micturition frequencies and decreased mean void volumes of Pirt −/− mice indicate that Pirt deficiency causes bladder overactivity. Interestingly, these changes in bladder function indicators are opposite to those of P2X3-null mice [11] . 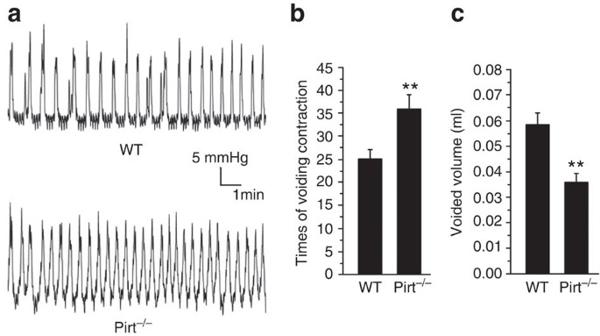Figure 1:Pirtdeficiency causes bladder overactivity. WT: WT mice.Pirt−/−:PirtKO mice. (a) The sample traces of cystometry recordings. (b) The histogram of voiding contraction times in 15 min. **P<0.01, two-tailed unpaired Student’st-test,n=6. (c) The histogram of the voided volume. **P<0.01, two-tailed unpaired Student’st-test,n=6. Error bars represent s.e.m. Figure 1: Pirt deficiency causes bladder overactivity. WT: WT mice. Pirt −/− : Pirt KO mice. ( a ) The sample traces of cystometry recordings. ( b ) The histogram of voiding contraction times in 15 min. ** P <0.01, two-tailed unpaired Student’s t -test, n =6. ( c ) The histogram of the voided volume. ** P <0.01, two-tailed unpaired Student’s t -test, n =6. Error bars represent s.e.m. Full size image Pirt and P2X3 are co-expressed in bladder nerve fibres The excitability of nerve fibres and smooth muscles within the bladder controls the contraction pattern. To understand the mechanism of voiding dysfunction, we examined the expression of Pirt in the bladder. The Tuj-1 antibody was used to detect nerve fibres, which are distributed in the urothelium, suburothelium and smooth muscle layers, and the antibody against smooth muscle actin (SMA) was used as smooth muscle marker. Pirt immunoreactivity (ir) occurred in a linear style and was co-localized with Tuj-1-ir ( Fig. 2a–c ). However, Pirt-ir was not expressed with SMA-ir ( Fig. 2d–f ). These results show that Pirt is expressed predominantly in nerve fibres of the bladder but not in smooth muscles. These data are consistent with the previous finding that Pirt is expressed specifically in almost all dorsal root ganglion (DRG) neurons including all of the non-peptide C-fibres [12] . 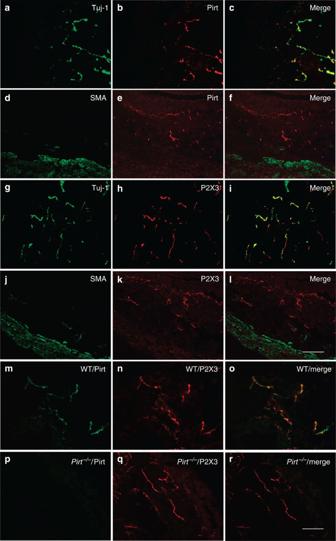Figure 2: Pirt and P2X3 are co-expressed in bladder nerve fibres. (a–l) The expression of Pirt and P2X3 in bladders. (a–c) Tuj-1-ir (green) and Pirt-ir (red) in the mouse bladder. (d–f) SMA-ir (green) and Pirt-ir (red) in the mouse bladder. (g–l) Tuj-1-ir (green) or SMA-ir (green) and P2X3-ir (red) in the mouse bladder. The corresponding merged images are on the right. Scale bar, 100 μm. (m–r) The co-expression of Pirt and P2X3. WT, WT mouse.Pirt−/−,Pirt-knockout mouse. Pirt-ir, green; P2X3-ir, red. The merged images are from the left-side images. Scale bar, 100 μm. Figure 2: Pirt and P2X3 are co-expressed in bladder nerve fibres. ( a – l ) The expression of Pirt and P2X3 in bladders. ( a – c ) Tuj-1-ir (green) and Pirt-ir (red) in the mouse bladder. ( d – f ) SMA-ir (green) and Pirt-ir (red) in the mouse bladder. ( g – l ) Tuj-1-ir (green) or SMA-ir (green) and P2X3-ir (red) in the mouse bladder. The corresponding merged images are on the right. Scale bar, 100 μm. ( m – r ) The co-expression of Pirt and P2X3. WT, WT mouse. Pirt −/− , Pirt -knockout mouse. Pirt-ir, green; P2X3-ir, red. The merged images are from the left-side images. Scale bar, 100 μm. Full size image Because P2X3-null mice also had decreased micturition frequencies [11] , we examined the expression of P2X3 in the bladder. P2X 3 -ir co-localized with Tuj-1-ir but not SMA-ir ( Fig. 2g–l ). This result is consistent with the report that P2X3 receptors were primarily expressed in bladder nerves [14] . Importantly, Pirt-ir was shown to co-exist with P2X3-ir in nerve fibres ( Fig. 2m–o ). Moreover, in Pirt null bladder, there were no significant changes observed in the P2X3-ir distribution ( Fig. 2p–r ). We also examined the expression of Pirt in DRG tissues. Immunohistochemistry results showed that the fluorescence signals of Pirt were widely expressed in DRG neurons consistent with the previous finding [12] , while the signals of P2X3 were relatively restricted in middle and small DRG neurons. Pirt and P2X3 are co-localized in many DRG neurons ( Supplementary Fig. 1 ). Pirt interacts with P2X3 to inhibit its activity Because both Pirt and P2X3 are co-expressed in bladder nerve fibres, we next determined whether Pirt interacts with P2X3. Pirt and P2X3, along with corresponding fusion labels, were transfected into HEK293T cells; the cells were then processed for co-immunoprecipitation. As shown in Fig. 3a , Pirt co-immunoprecipitates with P2X3 and vice versa. These results demonstrate that Pirt can interact with P2X3. 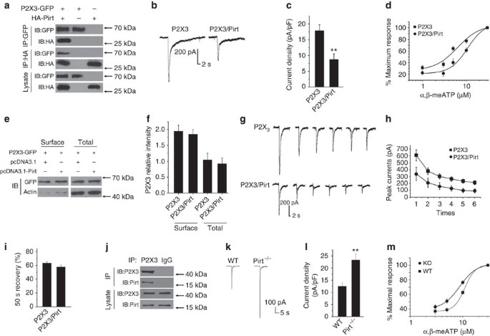Figure 3: Pirt interacts with P2X3 to inhibit its activity. The HEK293T cells were transfected as indicated. (a) The co-immunoprecipitation of Pirt and P2X3 in HEK293T cells. (b) The sample traces of inward currents induced by 10 μM α,β-meATP in HEK293T cells. (c) The histogram of P2X3 current density. **P<0.01, two-tailed unpaired Student’st-test,n=38. (d) The concentration–response curves for α,β-meATP-elicited currents in HEK293T cells. The smooth lines show the values predicted by a sigmoidal fit.n=12 for each concentration. (e) An example of an immunoblot obtained from the biotinylation assays. (f) The total protein level and cell surface expression of P2X3 in HEK293T cells was not altered by Pirt. The data were acquired from three individual experiments. (g) The sample traces of inward currents. Ten micromole α,β-meATP was applied six times with 50-s intervals for each time. (h) The plotting of P2X3 peak currents,n=38. (i) The histogram of P2X3 peak current recovery after 50-s intervals (the peak current induced by the second 10 μM α,β-meATP application/the first 10 μM α,β-meATP application).P>0.05, two-tailed unpaired Student’st-test,n=38. (j) Co-immunoprecipitation of Pirt and P2X3 in DRG neurons from WT mice. (k) The sample traces of inward currents induced by 30 μM α,β-meATP in neurons from WT mice orPirtKO (Pirt−/−) mice. (l) The histogram of the current densities of P2X3. **P<0.01, two-tailed unpaired Student’st-test,n=10. (m) The concentration–response curves for α,β-meATP-elicited currents in DRG neurons. The smooth lines show the values predicted by a sigmoidal fit;n=12 for each concentration. Error bars represent s.e.m. Figure 3: Pirt interacts with P2X3 to inhibit its activity. The HEK293T cells were transfected as indicated. ( a ) The co-immunoprecipitation of Pirt and P2X3 in HEK293T cells. ( b ) The sample traces of inward currents induced by 10 μM α,β-meATP in HEK293T cells. ( c ) The histogram of P2X3 current density. ** P <0.01, two-tailed unpaired Student’s t -test, n =38. ( d ) The concentration–response curves for α,β-meATP-elicited currents in HEK293T cells. The smooth lines show the values predicted by a sigmoidal fit. n =12 for each concentration. ( e ) An example of an immunoblot obtained from the biotinylation assays. ( f ) The total protein level and cell surface expression of P2X3 in HEK293T cells was not altered by Pirt. The data were acquired from three individual experiments. ( g ) The sample traces of inward currents. Ten micromole α,β-meATP was applied six times with 50-s intervals for each time. ( h ) The plotting of P2X3 peak currents, n =38. ( i ) The histogram of P2X3 peak current recovery after 50-s intervals (the peak current induced by the second 10 μM α,β-meATP application/the first 10 μM α,β-meATP application). P >0.05, two-tailed unpaired Student’s t -test, n =38. ( j ) Co-immunoprecipitation of Pirt and P2X3 in DRG neurons from WT mice. ( k ) The sample traces of inward currents induced by 30 μM α,β-meATP in neurons from WT mice or Pirt KO ( Pirt −/− ) mice. ( l ) The histogram of the current densities of P2X3. ** P <0.01, two-tailed unpaired Student’s t -test, n =10. ( m ) The concentration–response curves for α,β-meATP-elicited currents in DRG neurons. The smooth lines show the values predicted by a sigmoidal fit; n =12 for each concentration. Error bars represent s.e.m. Full size image To determine whether Pirt can modulate P2X3 activity, we measured the peak current densities of P2X3 transfected with Pirt in HEK293T cells. Compared with the control, the peak current density of P2X3 was significantly reduced in the presence of Pirt ( Fig. 3b,c ). Furthermore, we examined the concentration–response relationship for α,β-meATP activation. The HEK293T cells expressing P2X3 and Pirt showed an EC 50 value of 7.9 μM. In the HEK293T cells expressing only P2X3, the EC 50 value was 3.9 μM ( Fig. 3d ). However, the total protein levels and the cell surface expression of P2X3 in HEK293T cells were not altered by Pirt ( Fig. 3e,f ). If ATP or its selective agonist, α,β-meATP, is repeatedly applied to P2X3, the current amplitude of P2X3 has been shown to gradually decline [15] . Therefore, we also examined the effect of Pirt on the desensitization of P2X3 currents. In the presence of Pirt, P2X3 still showed characteristics of desensitization ( Fig. 3g,h ), and the decline of current amplitude did not differ significantly from that of the control ( Fig. 3i ). These results indicate that Pirt reduces the activity of P2X3 without altering its membrane expression and does not affect the desensitization of P2X3 currents. To test whether Pirt interacts with P2X3 in vivo , co-immunoprecipitation experiments were performed on tissues from the dorsal root ganglia (DRG). As shown in Fig. 3j , Pirt co-immunoprecipitates with P2X3 in the lysates of DRG tissues. To examine the P2X3 currents in DRG neurons of afferent nerves from the bladder of Pirt −/− mice or WT mice, we injected tetramethylindocarbocyanine perchlorate (DiI) into the bladders of mice. Three weeks later, the lumbosacral DRG neurons were dissociated, and the P2X3 currents in DRG neurons with DiI labelling were recorded. We found that DRG neurons from Pirt −/− mice had higher P2X3 current densities than those from WT littermates ( Fig. 3k,l ). Furthermore, we examined the concentration–response relationship for α,β-meATP activation in all neurons from lumbosacral (L6–S2) DRG (including non-bladder-innervating DRG neurons; Fig. 3m ). The WT neurons showed an EC 50 value of 7.96 μM. In Pirt KO neurons, the EC 50 value was 4.98 μM. Taken together, these results suggest that Pirt interacts with P2X3 in DRG neurons and that the deletion of Pirt causes P2X3 disinhibition. N-terminal 14 residues are necessary to inhibit P2X3 To map the critical region for Pirt to modulate P2X3 activity, we constructed a series of truncated mutants and transfected them with P2X3 into HEK293T cells. Electrophysiological recordings showed that the deletion of the entire amino-terminal (N-terminal) intracellular domain of Pirt (PirtΔN) eliminated its inhibition ability, while the deletion of the entire carboxyl-terminal intracellular domain of Pirt (PirtΔC) retained the inhibitory effect on P2X3 currents ( Fig. 4a,b ). These results indicated that the N-terminal intracellular domain is crucial for Pirt to reduce the activity of P2X3. Further analyses revealed that neither deletion of the amino-acid residue 2–26 of Pirt (PirtΔ(2–26)) nor deletion of the amino-acid residue 2–14 of Pirt (PirtΔ(2–14)) was capable of inhibiting P2X3 currents ( Fig. 4c,d ), suggesting that the N-terminal 14 amino-acid residues are necessary for Pirt to inhibit P2X3 activity. 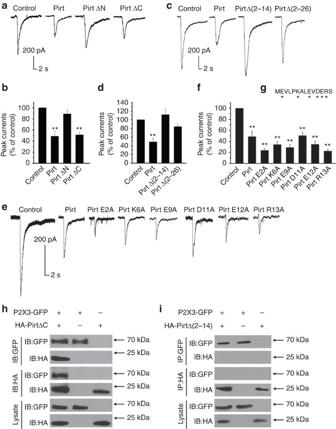Figure 4: N-terminal 14 amino-acid residues are necessary for Pirt to inhibit P2X3. The HEK293T cells were transfected as indicated. Control group cells were co-transfected with pcDNA3.1-P2X3 and pEGFP-N2. (a) The sample traces of inward currents induced by 10 μM α,β-meATP. (b) The histogram of the percentage of P2X3 peak currents. **P<0.01, versus control; one-way analysis of variance (ANOVA) and Tukeypost hocmeans comparisons.n=38. (c) The sample traces of inward currents induced by 10 μM α,β-meATP. (d) The histogram of the percentage of P2X3 peak currents. **P<0.01, versus control; one-way ANOVA and Tukeypost hocmeans comparisons.n=38. (e) The sample traces of inward currents induced by 10 μM α,β-meATP. (f) The histogram of the percentage of P2X3 peak currents. **P<0.01, versus control; one-way ANOVA and Tukeypost hocmeans comparisons.n=38. (g) Asterisks mark the charged amino acids in the N-terminal 14 amino-acid residues of Pirt. (h) PirtΔC forms a complex with P2X3 by co-immunoprecipitation assay in HEK293T cells transfected as indicated. (i) PirtΔ(2–14) does not form a complex with P2X3 by co-immunoprecipitation assay in HEK293T cells transfected as indicated. Error bars represent s.e.m. Figure 4: N-terminal 14 amino-acid residues are necessary for Pirt to inhibit P2X3. The HEK293T cells were transfected as indicated. Control group cells were co-transfected with pcDNA3.1-P2X3 and pEGFP-N2. ( a ) The sample traces of inward currents induced by 10 μM α,β-meATP. ( b ) The histogram of the percentage of P2X3 peak currents. ** P <0.01, versus control; one-way analysis of variance (ANOVA) and Tukey post hoc means comparisons. n =38. ( c ) The sample traces of inward currents induced by 10 μM α,β-meATP. ( d ) The histogram of the percentage of P2X3 peak currents. ** P <0.01, versus control; one-way ANOVA and Tukey post hoc means comparisons. n =38. ( e ) The sample traces of inward currents induced by 10 μM α,β-meATP. ( f ) The histogram of the percentage of P2X3 peak currents. ** P <0.01, versus control; one-way ANOVA and Tukey post hoc means comparisons. n =38. ( g ) Asterisks mark the charged amino acids in the N-terminal 14 amino-acid residues of Pirt. ( h ) PirtΔC forms a complex with P2X3 by co-immunoprecipitation assay in HEK293T cells transfected as indicated. ( i ) PirtΔ(2–14) does not form a complex with P2X3 by co-immunoprecipitation assay in HEK293T cells transfected as indicated. Error bars represent s.e.m. Full size image Because nearly half of the N-terminal 14 amino-acid residues are charged ( Fig. 4g ), we next used a targeted mutagenesis approach to determine whether these charged amino acids contribute to the inhibitory effect. A series of mutants with single charged amino acids substituted by alanine were constructed. However, all of these mutants were able to inhibit P2X3 currents ( Fig. 4e,f ), suggesting that there is a sophisticated interaction between Pirt and P2X3. To further confirm that the N-terminal 14 amino-acid residues is the key region for Pirt to bind with P2X3, we performed co-immunoprecipitation analysis and revealed that PirtΔC still interacted with P2X3 ( Fig. 4h ) while PirtΔ(2–14) did not ( Fig. 4i ). Taken together, these results suggest that the N-terminal 14 amino-acid residues are necessary for Pirt to interact with P2X3 to inhibit its activity. Pirt N14 inhibits P2X3 and alleviates bladder overactivity We next tested whether the peptide derived from the N terminus of Pirt could inhibit P2X3 activity. A Pirt N14 peptide with an intracellular delivery property was prepared by the fusion of the TAT peptide [16] at its C terminus. We performed competition assays in which the Pirt N14 peptide was incubated at different concentrations with cell lysates from HEK293T cells transfected with P2X3-GFP (green fluorescent protein) and HA-Pirt before immunoprecipitation. Our results revealed a dose-dependent reduction of Pirt bound to the P2X3 complex with an increased concentration of Pirt N14 peptide ( Fig. 5a ). The relationship between the concentration of the Pirt N14 peptide and the relative intensity of P2X3-GFP bands was fit by a single exponential function ( Fig. 5b ). These results implied that the Pirt N14 peptide could interrupt the interaction of P2X3 and Pirt by competitive binding. 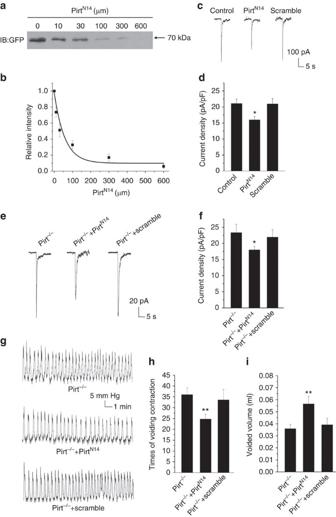Figure 5: PirtN14peptide inhibited P2X3 and alleviated the bladder overactivity ofPirt−/−mice. (a) An example of an immunoblot obtained from competition assays. (b) A dose-dependence curve was obtained after fitting a single exponential decay curve to the relative intensities obtained for the immunoblot bands;n=4 independent experiments. (c,d) The HEK293T cells expressing P2X3 were preincubated with 10 μM PirtN14peptide (PirtN14group), 10 μM scrambled peptide (scramble group) or buffer (control group) for 1 h. (c) The sample traces of inward currents induced by 10 μM α,β-meATP. (d) The histogram of the current densities of P2X3. *P<0.05, versus control; one-way analysis of variance (ANOVA) and Tukeypost hocmeans comparisons.n=30. (e,f) The acute dissociated lumbosacral DRG neurons fromPirtKO mice were preincubated with 10 μM PirtN14peptide (Pirt−/−+PirtN14), 10 μM scrambled peptide (Pirt−/−+scramble) or buffer (Pirt−/−) for 1 h. (e) The sample traces of inward currents induced by 30 μM α,β-meATP for 2 s in DRG neurons with DiI fluorescence. (f) The histogram of the current densities of P2X3. *P<0.05, versusPirt−/−; one-way ANOVA and Tukeypost hocmeans comparisons.n=10. (g) The sample traces of cystometry recordings. PirtN14or scrambled peptides were applied at a dosage of 20 mg kg−1. (h) The histogram of the voiding contraction times in 15 min. **P<0.01, versusPirt−/−; one-way ANOVA and Tukeypost hocmeans comparisons.n=7. (i) The histogram of the voided volume. **P<0.01, versusPirt−/−; one-way ANOVA and Tukeypost hocmeans comparisons.n=6. Error bars represent s.e.m. Figure 5: Pirt N14 peptide inhibited P2X3 and alleviated the bladder overactivity of Pirt −/− mice. ( a ) An example of an immunoblot obtained from competition assays. ( b ) A dose-dependence curve was obtained after fitting a single exponential decay curve to the relative intensities obtained for the immunoblot bands; n =4 independent experiments. ( c , d ) The HEK293T cells expressing P2X3 were preincubated with 10 μM Pirt N14 peptide (Pirt N14 group), 10 μM scrambled peptide (scramble group) or buffer (control group) for 1 h. ( c ) The sample traces of inward currents induced by 10 μM α,β-meATP. ( d ) The histogram of the current densities of P2X3. * P <0.05, versus control; one-way analysis of variance (ANOVA) and Tukey post hoc means comparisons. n =30. ( e , f ) The acute dissociated lumbosacral DRG neurons from Pirt KO mice were preincubated with 10 μM Pirt N14 peptide ( Pirt −/− +Pirt N14 ), 10 μM scrambled peptide ( Pirt −/− +scramble) or buffer ( Pirt −/− ) for 1 h. ( e ) The sample traces of inward currents induced by 30 μM α,β-meATP for 2 s in DRG neurons with DiI fluorescence. ( f ) The histogram of the current densities of P2X3. * P <0.05, versus Pirt −/− ; one-way ANOVA and Tukey post hoc means comparisons. n =10. ( g ) The sample traces of cystometry recordings. Pirt N14 or scrambled peptides were applied at a dosage of 20 mg kg −1 . ( h ) The histogram of the voiding contraction times in 15 min. ** P <0.01, versus Pirt −/− ; one-way ANOVA and Tukey post hoc means comparisons. n =7. ( i ) The histogram of the voided volume. ** P <0.01, versus Pirt −/− ; one-way ANOVA and Tukey post hoc means comparisons. n =6. Error bars represent s.e.m. Full size image To examine the effects of the Pirt N14 peptide on P2X3, we incubated the HEK293T cells transfected with P2X3 with Pirt N14 peptide or scrambled peptide for 1 h before electrophysiological recordings. The data showed that the Pirt N14 peptide significantly inhibited P2X3 current density, while scrambled peptide did not ( Fig. 5c,d ; Supplementary Fig. 2 ). These results further support that the Pirt N14 peptide is sufficient to inhibit P2X3 currents. Pirt −/− mice have a higher frequency of bladder voiding contractions ( Fig. 1a,b ), and DRG neurons from Pirt −/− mice had higher P2X3 currents than those from WT littermate mice ( Fig. 3k,l ). However, Pirt knockout does not influence the expression pattern of P2X3 ( Fig. 2p–r ). Therefore, we supposed that the bladder voiding dysfunctions might be due to P2X3 hyperactivity and a lack of Pirt regulation. To test whether Pirt supplementation could reduce the hyperactivity of P2X3 and alleviate the bladder overactivity of Pirt −/− mice, we performed electrophysiological recordings and urination behaviour experiments using Pirt −/− mice and the Pirt N14 peptide. We found that the currents of DRG neurons from Pirt −/− mice were significantly inhibited by Pirt N14 peptide treatment, while the scrambled peptide had no such effect ( Fig. 5e,f ). To test the Pirt N14 peptide transduction capability, we incubated the bladders of Pirt −/− mice with 60 mg kg −1 TAMRA-Pirt N14 (fluorescent-labelled TAT peptides, 5′-TAMRA-Pirt N14 -TAT-3′) for 30 min, cut them off and performed immunohistochemistry experiment ( Supplementary Fig. 3 ). We found that fluorescence signals of TAMRA-Pirt N14 showed a gradual weakening from the cavity side to the out side. The signals can be detected until deep into the muscle layer ( Supplementary Fig. 3a–c ). In the tissues of Pirt −/− bladder, the signals of TAMRA-Pirt N14 overlapped with the GFP signals of Pirt-expressing neural fibres ( Supplementary Fig. 3d–f ). These results suggested that Pirt N14 peptide can reach the neural fibres terminals beneath the suburothelial layer and might influence their activity. To examine urination behaviour, the Pirt N14 peptide was injected into the bladder cavity of Pirt −/− mice and incubated for 30 min. As shown in Fig. 5g–i , micturition frequencies were reduced, and the voided volume levels were elevated after Pirt N14 peptide treatment. We got the similar results in the Pirt −/− mice incubated with TAMRA-Pirt N14 ( Supplementary Fig. 4b,c,f ). To investigate whether the Pirt N14 peptide lose its inhibitory effect on bladder hyperactivity after P2X3 inhibition, we used A317491 to inhibit the P2X3 receptors. A317491 significantly decreased bladder voiding contraction times in Pirt −/− mice, but additional treatment of Pirt N14 failed to further decrease bladder voiding contraction ( Supplementary Fig. 5a,b ). These results demonstrate that the Pirt N14 peptide can inhibit the hyperactivity of P2X3 in the afferent neurons in the bladder and alleviate bladder overactivity in Pirt −/− mice. Role of Pirt in the bladder dysfunction of CYP-treated mice Clinically, there are many diseases that have urinary urgency and frequency symptoms, such as neurogenic bladder, overactive bladder, bladder outlet obstruction and interstitial cystitis [17] . It is very important to investigate whether Pirt is involved in the modulation of bladder activity. Therefore, we examined the role of Pirt in mice treated with cyclophosphamide (CYP), which has been used as a chemical irritant (via conversion to acrolein) in models of bladder overactivity [1] , [18] , [19] . CYP was intraperitoneal administered at the first, the third and the fifth day individually. After the administration, the bladder wall displayed macroscopic oedema and subcapsular vasculature were congested ( Supplementary Fig. 6 ), which is consistent with a previous report [20] . Immunohistochemistry results showed that Pirt-ir and P2X3-ir occurred predominantly in the nerve fibres of the bladder ( Fig. 6a ). We further quantified the amount of protein in whole bladders by western blot. There was no statistically significant difference in the expression of P2X3 between the CYP-treated bladders and the control bladders ( Fig. 6b,c ). However, the level of Pirt expression from CYP-treated bladders was much lower than the level from control bladders ( Fig. 6b,d ), suggesting that CYP-induced cystitis decreased the expression of Pirt. Through the quantitative PCR and western blot experiments with DRG tissues from mice treated with saline or CYP, We found that the relative amount of Pirt RNA ( Supplementary Fig. 7a ) and the mass of Pirt protein ( Supplementary Fig. 7b,c ) was not significantly changed in DRG tissues from CYP-treated mice. 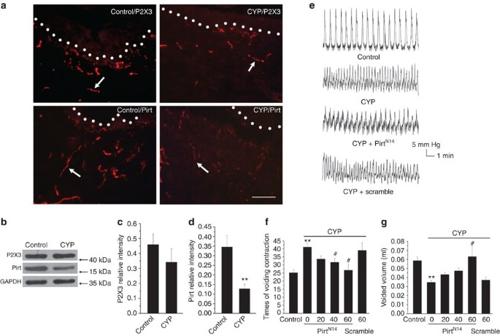Figure 6: The pathological role of Pirt in bladder dysfunction. (a) Expression of Pirt and P2X3 in the bladders of mice with or without CYP treatment. The portion above the dotted line is the urothelium, and the portion below is the suburothelial layer. The arrows indicate the nerve fibres with Pirt-ir or P2X3-ir. Scale bar, 50 μm. (b) Immunoblots of P2X3 and Pirt in bladder tissue lysates with GAPDH as the loading control. (c,d) The histogram of the relative expression of P2X3 and Pirt. **P<0.01, two-tailed unpaired Student’st-test,n=4 independent experiments. (e) The sample traces of cystometry recordings. PirtN14and scrambled peptide were administered at a dosage of 60 mg kg−1. Control: mice treated with saline. (f) The histogram of the voiding contraction times in 15 min. **P<0.01, versus control; two-tailed unpaired Student’st-test,n=10.#P40versus0<0.05, one-way analysis of variance (ANOVA) and Tukeypost hocmeans comparisons.n=7.#P60versus0<0.05, one-way ANOVA and Tukeypost hocmeans comparisons.n=8. (g) The histogram of the voided volume. **P<0.01, versus control; two-tailed unpaired Student’st-test,n=10.#P60versus0<0.05, one-way ANOVA and Tukeypost hocmeans comparisons.n=6. Error bars represent s.e.m. Figure 6: The pathological role of Pirt in bladder dysfunction. ( a ) Expression of Pirt and P2X3 in the bladders of mice with or without CYP treatment. The portion above the dotted line is the urothelium, and the portion below is the suburothelial layer. The arrows indicate the nerve fibres with Pirt-ir or P2X3-ir. Scale bar, 50 μm. ( b ) Immunoblots of P2X3 and Pirt in bladder tissue lysates with GAPDH as the loading control. ( c , d ) The histogram of the relative expression of P2X3 and Pirt. ** P <0.01, two-tailed unpaired Student’s t -test, n =4 independent experiments. ( e ) The sample traces of cystometry recordings. Pirt N14 and scrambled peptide were administered at a dosage of 60 mg kg −1 . Control: mice treated with saline. ( f ) The histogram of the voiding contraction times in 15 min. ** P <0.01, versus control; two-tailed unpaired Student’s t -test, n =10. # P 40 versus 0 <0.05, one-way analysis of variance (ANOVA) and Tukey post hoc means comparisons. n =7. # P 60 versus 0 <0.05, one-way ANOVA and Tukey post hoc means comparisons. n =8. ( g ) The histogram of the voided volume. ** P <0.01, versus control; two-tailed unpaired Student’s t -test, n =10. # P 60 versus 0 <0.05, one-way ANOVA and Tukey post hoc means comparisons. n =6. Error bars represent s.e.m. Full size image Our bladder function analysis data showed that the lowered expression of Pirt in CYP-treated bladders was accompanied by higher micturition frequencies and smaller voided volume compared with control group bladders ( Fig. 6e–g ). This dysfunction is quite similar to that of the Pirt −/− mice bladders. Because Pirt N14 peptides were able to alleviate the bladder overactivity of Pirt −/− mice, we next tested whether this peptide was also beneficial for the treatment of CYP-induced bladder dysfunction. As shown in Fig. 6e , the times of voiding contractions were reduced, and the voided volumes were increased when Pirt N14 peptides were applied, showing a concentration-dependent effect. TAMRA-Pirt N14 penetrated deep into the muscle layer ( Supplementary Fig. 3g–i ) and also reduced the times of voiding contractions ( Supplementary Fig. 4d–f ). Furthermore, we used A317491 to inhibit the P2X3 receptors, and A317491 significantly decreased bladder voiding contraction times of CYP mice. But additional treatment of Pirt N14 failed to further decrease bladder voiding contraction ( Supplementary Fig. 5c,d ). Taken together, these results indicate that Pirt has a pathological role in the bladder dysfunction of CYP-treated mice and a peptide derived from Pirt has inhibiting effects on bladder overactivity. Many diseases, such as interstitial cystitis, neurogenic bladder and bladder outlet obstruction, have common symptoms of urgency, micturition frequency and nocturia. The increased sensitization of C-fibre afferents is thought to play a key role in symptoms of bladder overactivity [21] . C-type fibres are distributed in the detrusor muscle, the lamina propria and close to the urothelium. These fibres express many receptors (for example, TRPV1, TRPA1, P2X3, TrkA and so on) that respond to various mediators released during inflammation, injury and ischaemia from a number of cell types [22] . The activation of these receptors increases the sensitization of C-fibre afferents. ATP was the first neurotransmitter reported to be released from the urothelium and can activate P2X3 receptors on nearby afferent nerve fibres [22] . It has been shown that pathology results in the augmented release of ATP from the urothelium, which can enhance the excitability of nearby bladder nerves [22] . P2X3-null mice exhibit a marked urinary bladder hyporeflexia, characterized by decreased voiding frequency and increased bladder capacity [11] . Moreover, Tempest et al . [23] have reported that P2X3 subunit expression changed greatly in patients with interstitial cystitis. Thus, P2X3 signalling is very important in the regulation of bladder function. In this study, Pirt, a small transmembrane protein, was found to contribute to the maintenance of the normal frequency of bladder voiding contractions and voided volume through modulating P2X3 in the bladder nerve fibres. We observed that a Pirt deficit caused bladder overactivity, as increased micturition frequencies and decreased mean void volumes were displayed in Pirt −/− mice. If we slowed down the infusion rate, we observed similar phenomena ( Supplementary Fig. 4 ). Pirt is restricted to the peripheral nervous system (predominantly DRG and trigeminal ganglia) [12] . In keeping with this observation, we found that Pirt is only expressed in bladder nerve fibres but not in detrusor smooth muscle cells, suggesting that Pirt may regulate the excitability of nerve fibres within the bladder to control the contraction pattern. The co-localization of P2X3 and Pirt in bladder nerve fibres provides further possibility for Pirt to regulate P2X3 activation and thereby to modulate bladder functioning. Indeed, whole-cell recordings from P2X3-expressing HEK293T cells showed that Pirt inhibited P2X3-mediated currents. Meanwhile, the density of inward currents induced by α,β-meATP from Pirt −/− DRG neurons was much higher than the density of currents from WT neurons. These results demonstrate that Pirt has the ability to negatively regulate P2X3 activity. Pirt physically interacts with TRPV1 and functions as a regulatory subunit of the TRPV1 complex [12] . The C terminus of Pirt binds to TRPV1 and several phosphoinositides, including phosphatidylinositol-4,5-bisphosphate. In addition, the enhancement of TRPV1 by phosphatidylinositol-4,5-bisphosphate requires Pirt. In the present study, by truncation analysis, the N-terminal intracellular domain of Pirt was identified as necessary for Pirt to inhibit P2X3. The interaction region was further limited to the first 14 amino acids of Pirt, which is completely different from the region of Pirt that regulates TRPV1. These results suggest that distinct regions of Pirt participate in the modulation of different channels. Because the N-terminal intracellular domain of Pirt has been confirmed to not bind to phosphoinositides [12] , it does not seem likely that Pirt modulates P2X3 via interacting with phosphoinositides. As a matter of fact, the Pirt N14 peptide competitively interrupted the interaction between Pirt and P2X3 and was sufficient to inhibit the P2X3 current in bladder DRG neurons, suggesting a direct binding mechanism for Pirt to modulate P2X3 activation. There are many charged amino-acid residues (6 out of 14) within the key N-terminal segment of Pirt. However, our alanine-scanning analysis excluded the possibility that any single amino acid determines the overall inhibition mechanism. So far, the crystal structure of the P2X4 ion channel in the closed state and in the ATP bounded open state has been resolved [24] , [25] . However, little information is available about the structure of the intracellular domains of P2X channels. A structural biology study of P2X3 and Pirt would be of much benefit to understand the mechanism underlying the P2X3 inhibition by Pirt. During the study of the DRG neuron currents, we found some currents were very slow to desensitize, which seemed like from P2X2/3, or even P2X2. And these currents were also inhibited to certain degree by Pirt either ( Supplementary Fig. 8 ). It is highly possible and interesting that the interaction of Pirt with P2X2/3, and even with P2X2, may involve in the modulation of functions of midheaven internal organs. This needs a careful research in future. TRP families are also expressed in neuronal fibres innervating the bladder and urethra [26] . TRPV1, TRPM8 and TRPA1 are the major TRPs in bladder C-fibre afferents and participate in the micturition reflex via afferent-type and efferent-type signalling [27] . Usually, only TRPV1 and TRPA1 are depicted on the same C-fibre terminal, while TRPM8 is expressed in a separate subpopulation of cold-sensitive C-fibre terminals [27] . The C terminus of Pirt binds to TRPV1 and several phosphoinositides and can potentiate TRPV1 (ref. 12 ). Recently, Pirt was further recognized as an endogenous regulator of TRPM8, and its C terminus is required for TRPM8 modulation [13] . These results suggest that the modulation of TRPs by Pirt might contribute to the regulation of bladder functions. However, Pirt positively regulates TRPV1 and TRPM8, which is logically contradictory to the observation that Pirt −/− mice have an overactive bladder. If Pirt could positively regulate the signals of TRPV1 leading to desensitization of the afferents, when Pirt was knocked out, TRPV1 should regain its activity and larger TRPV1 currents should be recorded in Pirt −/− DRG neurons than in wide-type DRG neurons, but the fact is opposite [12] . Meanwhile, Pirt −/− mice show impaired behavioural responses to noxious heat, capsaicinand cold, which implied that the afferents were desensitized via TRPV1 (ref. 12 ) or TRPM8 (ref. 13 ) without Pirt. Therefore, it is not likely that Pirt regulates the signals of TRPV1 or TRPM8 leading to desensitization of the afferents. Furthemore, Pirt N14 peptide failed to influence the currents of TRPV1 or TRPM8 expressed in HEK293T cells ( Supplementary Fig. 5e–j ). Taking into account that the Pirt N14 peptide inhibited the overactivity of the bladder and lost this effect after P2X3 had been blocked by A317491, we believe that P2X3 is a more important target for bladder overactivity. On the other hand, although the P2X3 currents were inhibited by Pirt N14 peptides in a dose-dependent manner, the effective concentrations of peptides were relatively high. To get more effective peptide, a systematic structure–functional analysis and screening is greatly needed. Chronic bladder inflammatory conditions, such as interstitial cystitis, have obvious symptoms of an overactive bladder [28] . In pathological conditions, including interstitial cystitis and obstructed and neurogenic bladder, the purinergic component of parasympathetic cotransmission is greatly increased [29] . Bladder inflammation induced by CYP in rats sensitizes and increases P2X3 receptor function [30] . CYP-induced cystitis is a frequently used animal model [19] , [20] , [30] , [31] . CYP is an antineoplastic agent, and it is metabolized to acrolein by the liver [32] , [33] . CYP and acrolein are chemical irritants that directly damage the urothelium and other cells of the bladder, resulting in cystitis in patients or animals [32] , [33] . Accompanied by the behaviours associated with an overactive bladder, higher micturition frequencies and smaller bladder capacities, our immunohistochemistry and western blot results showed that the expression of Pirt greatly decreased after 1 week of CYP treatment. This result is similar in Pirt −/− mice when Pirt deficiency occurs with bladder overactivity. However, the data from quantitative PCR and western blot indicated that the relative amount of Pirt RNA and the mass of Pirt protein was not significantly changed in DRG tissues from CYP-treated mice. These results implied that the Pirt downregulation in CYP-treated bladder was not caused by transcriptional or translational change, and an axonal transport change might be involved. The finding that the Pirt N14 peptide interrupts the interaction between Pirt and P2X3 and thereby inhibits P2X3 activation in the bladder DRG neurons provides a practical way to modulate the bladder voiding function in vivo . After the administration of the Pirt N14 peptide, the frequency of bladder voiding contractions in Pirt −/− mice was decreased, and the voided volume was increased. Furthermore, Pirt N14 peptide also reduced the frequency of voiding bladder contractions and restored the voided volume of CYP-treated mice in a dose-dependent manner. As P2X3 has been reported to be expressed in urothelium [7] , Pirt N14 may also inhibit these receptors and modulate urothelium’s functions, such as the secretion of ATP. If the local ATP concentration decreased, the excitability of P2X3 on the afferent nerve fibres beneath the urothelium would decrease. Therefore, we cannot exclude the possibility that the effects of the peptide are exerted partly via the urothelium, although it is a relatively indirect pathway. However, our TAMRA-Pirt N14 experiments showed that Pirt N14 peptide could reach the neural fibres terminals beneath the suburothelial layer and have the direct potential to inhibited the activity of neural fibres. Thus, our results strongly suggest a pathological role of Pirt in bladder dysfunction as well as a peptide derived from Pirt has inhibiting effects on bladder overactivity. Animals and plasmids Female C57BL/6 mice were housed three to four per cage with free access to food and water. They were maintained on a 12-h/12-h light–dark cycle. All animal experiments were carried out in adherence with the National Institutes of Health Guidelines on the Use of Laboratory Animals and approved by the Second Military Medical University Committee on Animal Care. Female Pirt −/− mice and WT littermates with the C57BL/6 background were provided by Dr Zong-Xiang Tang at the Nanjing University of Chinese Medicine. When WT mice were used for comparison with Pirt -knockout mice, only littermates were chosen. Female 2–3-month-old mice were used for each experiment. Full-length rat Pirt and P2X3 complementary DNA (cDNA) were cloned from rat brain by reverse transcription–PCR. GFP-tagged P2X3 was constructed by subcloning the full-length P2X3 cDNA into a pEGFP-N2 vector (Clontech). HA-tagged Pirt and PirtΔ(2–14) were constructed by subcloning the full-length or truncated Pirt cDNA into the pCMV-HA vector (Clontech). Full-length P2X3 cDNA was also subcloned into pcDNA3.1 3.1/myc-His(−) A (Invitrogen). These plasmids were used for co-immunoprecipitation assays. Full-length rat Pirt cDNA in pcDNA3.1/myc-His(−)A (Invitrogen) was also used for the biotinylation assays with pEGFP-N2-P2X3. The mutations of rat Pirt were acquired by PCR from WT Pirt cDNA. The rat cDNA of Pirt or its mutations were subcloned into the pEGFP-N2 vector (Clontech). These plasmids were used for electrophysiological experiments. Immunohistochemistry Urinary bladders from mice were fixed and processed for immunohistochemistry [34] . The mice were anaesthetized using 10% chloral hydrate and perfused through the aorta with 0.9% NaCl solution and 4% paraformaldehyde in 0.1 mol l −1 phosphate buffer (pH 7.4). The bladders were dissected out and immersed in 4% paraformaldehyde in 0.1 M PBS (pH 7.2) for 2–4 h. Then, the bladders were transferred to 25% sucrose in PBS and kept in the solution until they sank to the bottom. Next, the bladders were rapidly frozen, cut (10 μm in thickness) with a Leica cryostat and mounted on gelatin-coated slides. The following primary antibodies were used: 1:200 goat anti-Pirt (Santa Cruz), 1:200 rabbit anti-P2X3 (Roche Bioscience), 1:400 mouse anti-actin (Santa Cruz) and 1:200 mouse anti-Tuj-1 (Promega). The preparations were incubated with the primary antibodies in antiserum dilution solution overnight at 4 °C. Subsequently, the preparations were incubated with 1:200 FITC- or 1:400 Cy3- conjugated IgG (FITC and Cy3 conjugated, donkey anti goat for Pirt; Cy3 conjugated, donkey anti-rabbit for P2X3; FITC conjugated, donkey anti-mouse for Tuj-1 and SMA) for 1 h to visualize target proteins. All staining procedures were carried out at room temperature, and all of the incubations were separated by three washes in PBS for 5 min each. Images were taken with a Nikon digital camera DXM1200 (Nikon, Japan) attached to a Nikon Eclipse E600 microscope (Nikon). Cell culture HEK293T cells (catalogue No.GNHu17, Cell Bank of China Academy of Sciences) were maintained in DMEM containing 10% fetal bovine serum, 1% penicillin–streptomycin at 37 °C and 5% CO 2 . For the transient transfection of HEK293T cells, Lipofectamine 2000 (Invitrogen) and a calcium phosphate reagent (Promega) were used according to the manufacturer’s protocol. For immunoprecipitation and immunoblotting assays, cells were cultured in 24-well or six-well culture plates. For patch-clamp experiments, cells were cultured on coverslips in culture plate wells. Immunoprecipitation and immunoblotting For the co-immunoprecipitation assay in HEK293T cells, P2X 3 -GFP and HA-Pirt or HA-PirtΔ(2–14) were co-transfected into HEK293T cells. After 48 h, the cells were harvested. The cells were washed twice with cold PBS, solubilized with ice-cold lysis buffer (50 mM Tris-HCl, pH 8.0, 1 mM EDTA, 150 mM NaCl, 0.5% sodium deoxycholate, 0.02% sodium azide, 1 mM NaF, 1 mM sodium vanadate, 1 mM phenylmethylsulfonyl fluoride, 1% Nonidet P-40, 1 mM dithiothreitol, 0.1% SDS, 2 μg ml −1 pepstatin, 2 μg ml −1 leupeptin and 2 μg ml −1 aprotinin) and incubated on ice for 20 min. Lysates were clarified by centrifugation at 11,200 g for 10 min at 4 °C. For the co-immunoprecipitation assay in DRG tissue, lumbosacral (L6–S2) DRG neurons were harvested from adult female C57BL mice. For the immunoblotting assay, whole bladders were isolated from adult female C57BL mice. Each tissue was homogenized using a pestle tissue grinder at low speed in solubilization buffer (25 mM HEPES-NaOH (pH 7.4), 125 mM potassium acetate, 5 mM MgCl 2 , 0.32 M sucrose and 1% Triton-X-100). Proteins solubilized from each mouse tissue homogenate were collected. The protein concentration of the supernatants from tissue homogenates or cell lysates was determined by the Bradford method. For immunoprecipitation, 500 μl of the supernatant was incubated with 5 μl of the precipitating antibody for 3 h at 4 °C under mild agitation. Protein G-agarose beads (Roche) were then added and incubated for 3 h. The immunoprecipitated samples were washed three times with lysis buffer, boiled for 3–5 min in sample-loading buffer, subjected to SDS–polyacrylamide gel electrophoresis (SDS–PAGE), immunoblotted with the corresponding antibodies and visualized with enhanced chemiluminescence (ECL, Pierce). The following antibodies were used: 1:1,000 monoclonal mouse anti-GFP (Roche), 1:100 rabbit anti-GFP (Abmart), 1:3,000 monoclonal mouse anti-HA (Sigma), 1:200 rabbit anti-HA (Sigma), 1:10,000 HRP-conjugated secondary antibody (Kangchen), 1:100 goat anti-Pirt (Santa Cruz), 1:1,000 rabbit anti-P2X 3 (Neuromics) and 1:10,000 anti-GAPDH (Kangchen). To show the original positions of tagged or native proteins of interest, we put the nitrocellulose membrane with the bands of prestained protein ladder under the X-ray film and scanned the film. These full scans of western blots are presented in Supplementary Fig. 9 . Biotinylation of cell surface proteins HEK293T cells were co-transfected with pEGFP-N2-P2X3 and pcDNA3.1 or pcDNA3.1-Pirt. After 48 h, the cells were incubated with 1 mg ml −1 EZ-Link Sulfo-NHS-LC-Biotin (Pierce) in PBS for 30 min at 4 °C. After quenching, the cells were lysed in RIPA buffer. The supernatant from the cell lysate was incubated with ImmunoPure Immobilized Streptavidin (Pierce) at 4 °C overnight. The proteins were eluted from the beads using SDS–PAGE sample buffer, and western blot analysis was performed using the anti-GFP (Roche) or anti-β-actin (Kangchen) antibody. Electrophysiological recordings P2X3 currents were recorded in whole-cell patch-clamp mode from transfected HEK293T cells or dissociated DRG neurons. The pipette solution contained 130 mM KCl, 1 mM CaCl 2 , 2 mM MgCl 2 , 10 mM EGTA and 10 mM HEPES. The pH was adjusted to 7.2 with KOH. The external solution contained 140 mM NaCl, 5 mM KCl, 2.5 mM CaCl 2 , 1 mM MgCl 2 , 10 mM glucose and 10 mM HEPES. The pH was adjusted to 7.4 with NaOH. The pipette resistance was 6–8 MΩ. Whole-cell, voltage-clamp recordings were performed at room temperature (21–24 °C) with a MultiClamp 700 A amplifier (Axon Instruments, Foster City, CA, USA). The membrane potential was held at −70 mV, and those with series resistance above 20 MΩ were rejected. Analogue signals were filtered at 2 kHz and sampled at 10 kHz. Drug solutions were delivered by an OCTAFLOW system (ALA Scientific Instruments, Westbury, NY, USA). α,β-meATP (30 μmol l −1 ) was applied for 2 s. One barrel was used to apply a drug-free solution to enable rapid termination of the drug application. Experiments were controlled by Clampex 8.1 software (Axon Instruments). For Pirt N14 peptide experiments, the cells were incubated with the peptide for 60 min, and the current data were acquired within 20 min. Concentration–response relationship analysis As α,β-meATP (over 30 μM) was applied repeatedly at an interval of 5 min, the evoked current dramatically ran down during the second application of agonist. To avoid the run-down, we applied α,β-meATP twice at an interval of 10 min. The first concentration applied was 3, 5 or 10 μM, and the second concentration applied was 30 μM. The peak current elicited by α,β-meATP from 3 to 30 μM was normalized to the response of the same cell to 30 μM α,β-meATP. The mean of the normalized response was calculated for each concentration applied. Bladder neuron labelling Bladder DRG neurons were retrograde tracer labelled [30] . In brief, the mouse was first gently patted to micturate to empty the bladder. Under 10% chloral hydrate anaesthesia (10 ml kg −1 , i.p. ), the bladder was surgically exposed (lower abdominal incision ∼ 1 cm in length), and 15 μl of 1,1′-dioctadecyl-3,3,3,3,ioctadecyl-lindocarbocyanine perchlorate (DiI(18); 100 mg in 2 ml dimethylsulphoxide; Molecular Probes, Eugene, OR) was injected into the bladder cavity using a 30-gauge needle across the bladder dome. Any visible leakage of DiI from the injection site was removed with a cotton swab. The incision was closed with a 4.0 silk suture, and the mice were allowed to recover. After surgery, the mice were deprived of water for 5 h. Three weeks later, DRG neurons were isolated and dissociated for electrophysiological recordings. DRG cell dissociation Mice were deeply anaesthetized with 10% chloral hydrate. Lumbosacral (L6–S2) DRG neurons were harvested for acute dissociation and whole-cell recordings. Ganglia were removed and immersed temporarily in Neurobasal medium (Gibco, Invitrogen, Grand Island, NY) over ice until all of the DRG neurons were harvested. Then, the DRG neurons were transferred to fresh Neurobasal medium containing B27 supplements (Gibco, Invitrogen, Grand Island, NY) and minced. The same volume of Neurobasal medium containing B27 supplements, collagenase (type 4; 4 mg ml −1 Worthington Biochemical, Lakewood, NJ) and trypsin (2 mg ml −1 ; Sango biotech, Shanghai, China) was added into the DRG tissue fragments. The tissue samples were mixed and incubated at 37 °C, 5% CO 2 for 60 min. After that, the DRG neurons were collected by centrifugation at 150 g for 5 min and washed three times with Neurobasal medium. Then, the DRG tissue fragments were resuspended in B27-supplemented, enzyme-free Neurobasal medium, pipetted 20 times and allowed to stand for 10 min. The cells in the supernatant were plated on poly- D -lysine-coated coverslips (Becton Dickinson Labware, Bedford, MA) and incubated at 37 °C, 5% CO 2 for 2–3 h before electrophysiological studies. Only neurons with DiI florescence were studied. All recordings were performed within 10 h after plating. Peptide competition assays Membrane-permeant Pirt N14 peptide (MEVLPKALEVDERSYGRKKRRQRRR), Pirt(1–14) amino-acid residues with a TAT tag, was synthesized by Shanghai Science Peptide Biological Technology Co. Ltd. Typically, 100–200 μl of the HEK293T cell lysates that were transfected with P2X3-GFP and HA-Pirt were incubated with different concentrations (0–600 μM) of the Pirt N14 peptide for 3 h at 4 °C. Then, immunoprecipitation was performed. Immunoprecipitates were detected by antibodies against GFP (Roche). Behavioural study The CYP animal model was induced by an intraperitoneal application of CYP (100 mg kg −1 ; Sigma) dissolved in 0.9% NaCl on days 0, 2 and 4; control mice received the solvent only. On day 5, cystometry was performed [35] . Mice were anaesthetized using 3% chloral hydrate (20 ml kg −1 , i.p.) and fixed on a board. A PE-10 polyethylene catheter (Anilab, Ningbo, Zhejiang, China) was inserted via a midline abdominal incision into the bladder through its dome. The intravesical catheter was connected via a three-way stopcock to a pressure transducer (Alcott Biotech Co., Ltd., Shanghai, China) and to a micro-infusion pump (Longer Precision Pump Co., Ltd., Baoding, China) for recording intravesical pressure and for infusing saline into the bladder, respectively. Intravesical pressure was continuously recorded using data acquisition software (Alcott Biotech Co., Ltd., Shanghai, China). After catheter implantation, mice were left undisturbed for ∼ 30 min for bladder stabilization. After this period, the tail was pinched, and the cystometry was performed if the mouse showed a flick reaction. Saline at 37 °C was infused at a rate of 0.1 ml min −1 . For the Pirt N14 peptide study, 200 μl of the peptide solution with corresponding concentration (20, 40 or 60 mg kg −1 ) was injected into the bladder cavity through the three-way stopcock. This volume of peptide solution swept away the saline in the catheter and bladder cavity and about 90 μl (WT or Pirt −/− mice) or 50 μl (CYP-treated mice) peptide solution was left in the cavity. After injection, the bladder was incubated for 30 min. How to cite this article: Gao, X.-F. et al . Pirt reduces bladder overactivity by inhibiting purinergic receptor P2X3. Nat. Commun. 6:7650 doi: 10.1038/ncomms8650 (2015).